An angular fluidic channel for prism-free surface-plasmon-assisted fluorescence capturing Surface plasmon excitation provides stronger enhancement of the fluorescence intensity and better sensitivity than other sensing approaches but requires optimal positioning of a prism to ensure optimum output of the incident light. Here we describe a simple, highly sensitive optical sensing system combining surface plasmon excitation and fluorescence to address this limitation. V-shaped fluidic channels are employed to mimic the functions of a prism, sensing plate, and flow channel in a single setup. Superior performance is demonstrated for different biomolecular recognition reactions on a self-assembled monolayer, and the sensitivity reaches 100 fM for biotin–streptavidin interactions. Using an antibody as a probe, we demonstrate the detection of intact influenza viruses at 0.2 HA units ml −1 levels. The convenient sensing system developed here has the advantages of being prism-free and requiring less sample (1–2 μl), making this platform suitable for use in situations requiring low sample volumes. Fluorescent labelling is a powerful tool for high-sensitivity detection of biomolecular interactions [1] , [2] , [3] , [4] , [5] . In particular, fluorescence is one of the most frequently used means of evaluating ligand–analyte complex formation in homogeneous and heterogeneous assays, as transduction of the target-binding event facilitated by fluorophores enables real-time monitoring [6] . Surface plasmon (SP) excitation is an appealing way to enhance the fluorescence intensity and sensitivity of the labelled products [7] , [8] , [9] , [10] , [11] , [12] , [13] . The SP phenomenon can be induced using a sensing plate composed of a thin metal film and a transparent substrate. When the SP is excited, an enhanced electric field appears in the vicinity of the metal surface (generally in a region less than ~1 μm from the surface). Then, if analytes conjugated with fluorescent tags are present in this electric field-enhanced region, their signal will be increased, resulting in a detection system with greater sensitivity. To excite the SP, the metal surface should be irradiated with p-polarized light at a certain incident angle from the substrate side. To this end, the Kretschmann configuration [14] is widely used, in which the transparent substrate of the sensing plate is attached to an optically matched prism. A flow channel is often set up using a polydimethylsiloxane (PDMS) spacer [12] , [15] , [16] on the metal film of the sensing plate, to help minimize the sample volume. The prism, sensing plate, and flow channel are discrete items, which need to be attached and detached in each independent experiment. This requires much more preparation time for the measurement, which decreases the usability. Furthermore, the optical setup is further complicated by the use of a prism, which has to be angled appropriately to ensure the optimum output of incident light. Therefore, such a system cannot function if misalignment due to vibration during carrying occurs. This, in turn, means the system is less portable. These facts limit the range of applications of SP-based sensing devices. Another approach to develop a prismless SP-assisted device has been reported in which a grating structure is used as a substitute for a prism [17] , [18] , [19] . However, such a sensing system also requires significantly complicated adjustment of the optical axis. Furthermore, the sensing plate and fluidic channels of the grating system are discrete, and evaluation of multiple samples is difficult. To overcome these issues, we introduce a V-shaped trench-sensing system, which combines the prism-like functionality, sensing plate and flow channel in a single setup. The use of this all-in-one setup on the sensor chip simplifies the measurement. As it is unnecessary to carefully adjust optical alignment, all we have to do is set the chip on the flat sample stage in our equipment. It also allows a sensing system based on SP-assisted fluorescence enhancement to be downsized, which will also contribute to cost reductions. Furthermore, by creating multiple spots immobilized with analyte-capture probes in one or more flow channels using a machine like an inkjet printer, in principle, multiple samples can be simultaneously measured in a single channel or on a piece of the chip [20] . Herein, we discuss the detailed design of a chip that can be used in situations requiring sensitive detection and can be extended to a wide range of biorecognition elements. V-trench chip and fluorescence imaging The chip used in this study has a size of 28 × 40 × 1.5 mm 3 , as displayed in Fig. 1a . The chip has four V-trench channels, which make it possible to conduct four independent detection tests simultaneously. The width of the upper opening and the length of the channels are 300 μm and 35 mm, respectively. Fluid reservoirs for injecting the solution are formed at the ends of the channels. The sizes and shapes of the reservoirs are shown in Supplementary Fig. S1 . 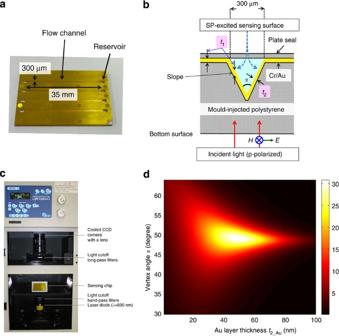Figure 1: Configuration of the sensing system. (a) Top view of the chip containing the fluidic channel. Sizes are indicated. (b) Cross-sectional image of the V-shaped channel. (c) Details of the detection system with a cooled CCD camera used in the present study, with the parts indicated. (d) Computer simulation of the electric field enhancement factor used to determine the most appropriate combination of Au-layer thickness and vertex angle of the V-trench for optimal sensitivity of the system. Figure 1b shows a cross-sectional image of the V-trench channels. The base chip used is mould-injected polystyrene (Cluster Technology, Higashi-Osaka, Japan). The tip of the trench is flat for easy fabrication, and an adhesive Cr film and an Au film for SP excitation are deposited on the chip using an evaporation system (R-dec, Tsukuba, Japan). Analytes with fluorescent conjugates are immobilized on the V-trench slopes by injecting them into the reservoirs and allowing them to flow to the channels by capillarity. When the analyte is flowing, the V-trenched channels are sealed with a plate seal to prevent flooding outside the channels. This sample preparation procedure is graphically explained in Supplementary Fig. S2 . Incident light propagates from the bottom of the chip. It irradiates the slope of the V-trench diagonally, so the slope of the V-trench channels mimics the function of the bottom surface of the regular prism in conventional SP-sensing (see Supplementary Fig. S3 ). In this way, the V-trench mimics the functions of a prism, sensing plane and flow channel. Furthermore, multiple-sample measurement is possible if multiple spots immobilized with analyte-capture probes are fabricated in a single channel or on a piece of the chip ( Supplementary Fig. S3 ), although such probes are formed on the whole surface of the sensing plane in the present experiment. The design of the vertex angle α and the Au-film thickness is discussed in detail below. Figure 1: Configuration of the sensing system. ( a ) Top view of the chip containing the fluidic channel. Sizes are indicated. ( b ) Cross-sectional image of the V-shaped channel. ( c ) Details of the detection system with a cooled CCD camera used in the present study, with the parts indicated. ( d ) Computer simulation of the electric field enhancement factor used to determine the most appropriate combination of Au-layer thickness and vertex angle of the V-trench for optimal sensitivity of the system. Full size image The optical system used involves a cooled CCD camera system for chemical-luminescence imaging (Light-Capture II, Atto, Tokyo, Japan) ( Fig. 1c ). We mounted a laser diode with a wavelength of 690 nm (Shibasaki, Chichibu, Japan) as a light source and irradiated the V-trench chip with p-polarized light to excite the SP ( Fig. 1b ). Band-pass filters (M.C. 680 and M.C. 690, Asahi Spectra, Tokyo, Japan) are placed between the laser and the chip to control the laser-light intensity. Fluorescence-conjugated analytes are detected by the cooled CCD camera system through three long-pass filters (HQ720LP, Chroma, Bellows Falls, VT, USA). Alexa Fluor 700 (Life Technologies, Carlsbad, CA, USA), with an excitation band at 702 nm and an emission band at 723 nm, was used as a fluorescent material. The camera exposure time was 120 s. In addition to Fig. 1c , a detailed schematic of the optical system is given in Supplementary Fig. S4 . Optimization of the Au thickness and V-trench vertex angle The electric-field amplitude was calculated using the finite-difference time-domain (FDTD) method to help with the chip design for appropriate SP excitation. P-polarized light with a wavelength of 690 nm is assumed to be used. In addition, it is assumed that the film thickness of the Cr or Au layer on the slope of the V-trenched channels is uniform, with vertical thickness t 1 and deposited thickness t 2 (perpendicular to the slope), as shown in Fig. 1b . In this case, the relationship between t 1 and t 2 for each layer is where α is the vertex angle of the V-trench. Furthermore, the polystyrene-based V-trench with deposited Cr, Au and buffer layers is assumed to be covered with water. The buffer layer is generally necessary to prevent fluorescence quenching due to energy transfer to the metal. The thickness t 1 of the adhering Cr is set to be 0.6 nm, which is the minimum thickness that we can control. Furthermore, the buffer layer is assumed to have a thickness t 2 of 20 nm. The complex refractive indices of polystyrene, Cr, Au, the buffer layer and water at a wavelength of 690 nm used in the calculation are 1.583 (ref. 21 ), 3.798+ i 4.369 (ref. 22 ), 0.1601+ i 3.816 (ref. 22 ), 1.45 and 1.329 (ref. 22 ), respectively. Based on these values, the electric field enhancement factor relative to that of the incident light at the surface of the buffer layer is calculated as a function of t 2_Au ( t 2 for the Au film) and α . Figure 1d shows the result of this simulation. It is found that the enhancement factor | E / E 0 | 2 reaches 31 when α =49° and t 2_Au =49 nm, where E is the electric-field intensity at the buffer layer surface and E 0 is that of incident light. In this case, t 1_Au ( t 1 for the Au film) is ~120 nm. These values were used in all subsequent experiments. Basic analysis of biomolecular interactions on biotin–SAM To elucidate the biosensing ability, we examined different types of ligand interactions in the analytes, such as, (i) the interactions of streptavidin and biotin, (ii) DNA–DNA hybridization and (iii) influenza virus detection using an anti-influenza antibody. Initially, we analysed biotin–streptavidin interactions, as shown in Fig. 2a . This is considered to be a high-affinity molecular interaction for biorecognition [23] . For specific analyses, the V-trench flow channels were tested using Alexa-Fluor-700-conjugated streptavidin in phosphate-buffered saline (PBS; pH 7.4; Wako Chemicals, Osaka, Japan) against biotin–SAM ( Fig. 2b ). 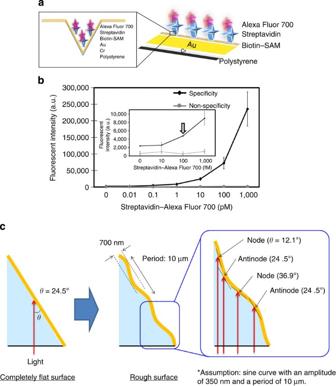Figure 2: Analyses of streptavidin interaction with biotin–SAM. (a) Diagrammatic representation of layers on the chip and biomolecular immobilization. The layers of the V-trenched fluidic channel are indicated. (b) Graphical representation of streptavidin and biotin interaction. Both specific and nonspecific reactions are shown. The arrow indicates the detection limit. The inset shows the values at femtomolar concentrations. The nonspecific reaction is a control measurement with fluorescent-labelled antibody and biotin interactions. Error values are calculated from five repetitions and are defined as the s.e.m. (c) Schematic image of the wavy V-shaped trench surface. Figure 2: Analyses of streptavidin interaction with biotin–SAM. ( a ) Diagrammatic representation of layers on the chip and biomolecular immobilization. The layers of the V-trenched fluidic channel are indicated. ( b ) Graphical representation of streptavidin and biotin interaction. Both specific and nonspecific reactions are shown. The arrow indicates the detection limit. The inset shows the values at femtomolar concentrations. The nonspecific reaction is a control measurement with fluorescent-labelled antibody and biotin interactions. Error values are calculated from five repetitions and are defined as the s.e.m. ( c ) Schematic image of the wavy V-shaped trench surface. Full size image To facilitate a clearer understanding of a typical measurement, a demonstration of the fluorescence observation is shown in the Supplementary Movie 1 . For simplicity, a solution of Alexa-Fluor-700-conjugated streptavidin was directly injected onto the V-trench surface for this movie, with immobilized biotin–SAM. As shown in Fig. 2b , when the streptavidin concentration reaches 100 fM, the signal intensity is enhanced by a factor of >2. Therefore, this was defined as the limit of detection. The signal intensity shows a twofold increase when the streptavidin concentration is increased 10-fold in the region below 1 pM. Thereafter, it increases by a factor of ~3 for the same streptavidin concentration increase. These increments were completely absent when Alexa-Fluor-700-conjugated anti-rabbit antibody was used on biotin–SAM as a control. In principle, the enhanced electric field resulting from SP excitation occurs when p-polarized light irradiates the surface. On the other hand, SP excitation does not occur under s-polarized light irradiation; weak evanescent fields only appear on the V-shaped trench surface under total reflection of the light, and the evanescent fields cause weak fluorescence from the tags. Thus, we measured the signal for s-polarized light (with the same incident light intensity for p-polarized light irradiation) as a reference system in which SP excitation does not appear. From this result, the size of the effect of the SP excitation was checked by comparing the signals for s- and p-polarized light. Note that in this analysis, we employed a V-trench chip with Cr, Au and SiO 2 ( t 1 =50 nm) layers, and Alexa-Fluor-700-conjugated streptavidin was attached directly to the SiO 2 surface. It was found that the signal obtained under s-polarized light was 7 times as weak as that obtained under p-polarized light. FDTD simulation showed that | E / E 0 | 2 for s-polarized light is ~7 × 10 −3 , whereas that for p-polarized light is ~31 ( Fig. 1d ). These calculations show that the signal theoretically differs by a factor of ~4,000, depending on the polarization. However, the actual value obtained was 7, as mentioned above. The gap between the experimental and theoretical results may be due to (i) the roughness of the V-trench surface, (ii) production tolerances in the thickness of the Au layer and the vertex angle of the V-trench and (iii) the fact that the flat tip of the V-trench, indicated in Fig. 1b and Supplementary Figs S1 and S3 , causes light leakage, resulting in fluorescence even under s-polarized light irradiation. Therefore, in turn, the signal intensity depends on these issues. Figure 1d indicates the precise dependences of the signal on the Au-layer thickness and the V-trench vertex angle. On the other hand, we can roughly estimate the influence of the roughness on the signal, as shown in Fig. 2c . This figure presents a schematic image of the wavy V-shaped trench surface. The shape of the V-trench surface is assumed to be sinusoidal, with an amplitude of 350 nm and a period of 10 μm. This roughness was determined by taking the manufacturer’s guarantee into account. If the surface is completely flat, the angle θ between the surface and incident light direction is 24.5°. However, θ has a wide angular range from 12.1° to 36.9° if the surface has such a roughness, and these angles correspond to V-shaped trench vertex angles α from 24.2° to 73.8°. This means that there are some regions where SP excitation hardly occurs on the V-shaped trench surface. This, in turn, indicates that the fluorescent signal also depends on the roughness. It is difficult to discuss the signal value quantitatively, as the roughness varies among the samples. However, it is clearly found that a low roughness contributes to a higher sensitivity. We further expanded the applications of the present sensing system to the diagnosis of DNA-duplex formation ( Fig. 3a ). To analyse this hybridization on biotin–SAM, a sandwich layer was formed using streptavidin and biotinylated dT 24 . Duplex formation was measured with paired (dA 20 ) and unpaired sequences (dT 20 ), as pairing will create a spacer region (dT 24 versus dA 20 ) for ideal complementation. The system detects the specific sequence (dA 20 ) at concentrations as low as 1 nM, whereas the dT 20 sequence does not show a significant fluorescent signal ( Fig. 3b ). 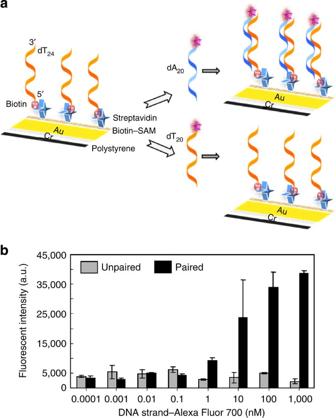Figure 3: Analyses of DNA-duplex formation on biotin–SAM. (a) To attach the molecules, a biotin–streptavidin–biotin sandwich was made. dT24was immobilized on the chip. Both pairing and nonpairing sequences were tested using dA20and dT20, respectively. (b) Fluorescent intensity as a function of the concentration of the DNA strand with Alexa Fluor 700. Error values are calculated from five repetitions and are defined as the s.e.m. Figure 3: Analyses of DNA-duplex formation on biotin–SAM. ( a ) To attach the molecules, a biotin–streptavidin–biotin sandwich was made. dT 24 was immobilized on the chip. Both pairing and nonpairing sequences were tested using dA 20 and dT 20 , respectively. ( b ) Fluorescent intensity as a function of the concentration of the DNA strand with Alexa Fluor 700. Error values are calculated from five repetitions and are defined as the s.e.m. Full size image Detection of influenza viruses We further tested the detection of the influenza virus using an antibody probe that was generated previously [24] . Influenza occurs all over the world, causing death and imposing severe burdens on human health and the economy. Developing detection systems is crucial and will prevent severe consequences [25] . Therefore, we used the present system for detection of an influenza strain. As an example influenza surveillance application, we tested a strain of A/Udorn/307/1972 (H3N2) supplied by Nihon University using the developed antibody [24] , hereafter referred to as the anti-A/Udorn/307/1972 antibody. For this experiment, a carboxylic-terminated (COOH)–SAM was used. After immobilization of the A/Udorn/307/1972 virus on the COOH surface, the anti-A/Udorn/307/1972 antibody (100 nM) was added, and then 10 nM Alexa-Fluor-700-conjugated anti-rabbit antibody (as a secondary antibody) was attached to the anti-A/Udorn/307/1972 antibody to induce fluorescence ( Fig. 4a ). As shown in Fig. 4b , the fluorescent signal increases logarithmically with increasing amounts of A/Udorn/307/1972 virus between 0.02 and 20 HA units ml −1 , after which it is saturated. The detection limit of A/Udorn/307/1972 was estimated to be 0.2 HA units ml −1 . 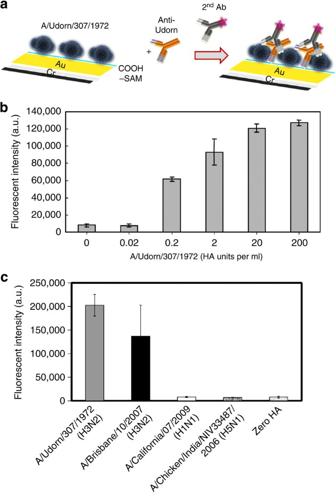Figure 4: Detection of influenza viruses. (a) Schematic representation of influenza virus detection. A/Udorn/307/1972 (H3N2) attached to the chip surface was detected using the anti-A/Udorn/307/1972 antibody and the Alexa-Fluor-700–labelled anti-rabbit antibody. (b) Sensitivity for A/Udorn/307/1972 (H3N2), showing a sensitivity level of 0.2 HA units per ml. (c) Detection of influenza strains H3N2 (A/Udorn/307/1972 and A/Brisbane/10/2007), and recombinant haemagglutinin from influenza H5N1 (A/chicken/India/NIV33487/2006) and H1N1 (A/California/07/2009) with 2,000 HA units per ml. The signal obtained for zero HA (the leftmost point inb) is also shown. Error values are calculated from five repetitions and are defined as the s.e.m. Figure 4: Detection of influenza viruses. ( a ) Schematic representation of influenza virus detection. A/Udorn/307/1972 (H3N2) attached to the chip surface was detected using the anti-A/Udorn/307/1972 antibody and the Alexa-Fluor-700–labelled anti-rabbit antibody. ( b ) Sensitivity for A/Udorn/307/1972 (H3N2), showing a sensitivity level of 0.2 HA units per ml. ( c ) Detection of influenza strains H3N2 (A/Udorn/307/1972 and A/Brisbane/10/2007), and recombinant haemagglutinin from influenza H5N1 (A/chicken/India/NIV33487/2006) and H1N1 (A/California/07/2009) with 2,000 HA units per ml. The signal obtained for zero HA (the leftmost point in b ) is also shown. Error values are calculated from five repetitions and are defined as the s.e.m. Full size image Analytical sensor systems for the diagnosis of infectious diseases are in high demand in recent years [26] , [27] , [28] , [29] . Previously, the NanoSign influenza A/B detection kit developed by Lee et al. [26] was shown to have a sensitivity of 1.13±0.11 HA units. Another sensing system was reported to have a sensitivity level of 0.013 HA units ml −1 for the detection of influenza viruses [27] . The sensitivity of our developed system was between these two results. The diameter of the influenza virus is considered to be ~100 nm. In the FDTD calculation, the value of | E / E 0 | 2 at a point 100 nm away from the V-trench surface is ~11, whereas | E / E 0 | 2 =31 at the surface of the trench. Thus, the large size of the virus may cause the fluorescence intensity to decay by ~65%. However, if the flatness of the V-shaped trench surface is improved, our system can achieve higher sensitivity, as mentioned above. Furthermore, the V-shaped fluidic channel has other benefits: an all-in-one structure, simple optical alignment and the possibility of concurrent measurement of multiple samples. In addition, our system has another interesting feature, in that the measurement is finished in only 2 min, whereas 30 min is required in the method reported by Wang et al. [27] Furthermore, although we used a cooled CCD camera for detection, the use of photodiodes for optical pickup on a CD, DVD or CMOS image sensor will allow significant downsizing of the system and reductions in the power requirements as well as the cost. Such a small imaging system will be highly useful for on-site measurements during outbreaks or for surveillance of pathogens. This work will be carried out as a next step. Recently, other sensing systems for biomolecular detection have been proposed, for example, a sensor utilizing localized SP resonance (LSPR) caused by Au nanostructures [30] , [31] . The sensitivity of our sensor system seems to be almost equivalent to that of the LSPR sensor, and the LSPR sensor does not have the benefits of our system, especially the all-in-one structure and the possibility of multiple-sample measurement. These facts also establish the significance of our sensing system. Finally, we further attempted to detect another influenza viral sample (A/Brisbane/10/2007 (H3N2)), as well as recombinant haemagglutinin from influenza H5N1 (A/chicken/India/NIV33487/2006) and H1N1 (A/California/07/2009) with 2000 HA units ml −1 against the Anti-A/Udorn/307/1972 antibody ( Fig. 4c ). The signal obtained for zero HA (the leftmost point in Fig. 4b ) is also shown in the figure. From this figure, it is clear that we successfully detected A/Brisbane/10/2007 (H3N2), whereas our system is insensitive to the remaining haemagglutinin. It is found that the antibody has affinity with H3N2 stains and does not recognize the other tested types. This newly designed fluorescence sensing system with V-trenched fluidic channels operates based on SP excitation, and it has the advantages of being a simple, prism-free analytical tool that requires very low sample volumes (1–2 μl). Calculations allowed the most appropriate combination of Au thickness and vertex angle of the V-trench to be determined. Furthermore, we have experimentally demonstrated the efficient performance of this system. The detection limit of fluorescent Alexa-Fluor-700-conjugated streptavidin and biotin-based interactions were determined to be 100 fM, whereas for influenza viruses, the detection limit was 0.2 HA unit ml −1 , which is comparable with those of other proposed sensitive detection systems. Moreover, the developed sensing system has additional advantages, including its suitability for a wide range of biomolecular interactions and its simplicity. The developed system has great potential from various viewpoints, and we believe it will be a leading candidate for next-generation biosensors. Analyses of biomolecular interactions on biotin–SAM The sensing surfaces were coated with an Au overlay using the evaporation method and were incubated with 0.1 mM of a biotin–SAM formation reagent (Dojindo Laboratories, Kumamoto, Japan) in absolute ethanolic solution for 3 h at room temperature with shaking. The biotin–SAM formed over the entire surfaces of the 35-mm-long channels. Next, this biotin-coated surface was washed thoroughly with copious volumes of ethanol and dried under N 2 gas. Then, a plate seal was attached to the chip. A total of 2 μl of streptavidin-conjugated Alexa-Fluor-700 in PBS was gradually injected into one flow channel through the reservoir, and the flow was stopped after the channel was filled. Another channel was used as the control, into which Alexa-Fluor-700-conjugated anti-rabbit antibody (Invitrogen, USA) was injected to determine the nonspecificity. These fluorescent samples varied in concentration from 10 fM to 1 nM. After 20 min of incubation at room temperature, the channels were thoroughly washed with PBS. The absolute value of the fluorescent signal was measured in a horizontally-long rectangular area of ~5 × 8 mm 2 in the channel (laser-light irradiated) region. Simultaneously, the value in a non-illuminated region (far enough from the channel) with the same area was measured. Each fluorescent intensity shown in Fig. 2b was obtained by subtracting the absolute value of the non-illuminated region from that of the channel region. Note that the fluorescent intensity was also obtained during injection of PBS not containing Alexa-Fluor-700 into the channel; the fluorescent intensities from this experiment are shown as the points at zero concentration on the x axis of Fig. 2b . Similarly, on the biotin–SAM surface, a sandwich layer was formed using streptavidin followed by biotinylated DNA (dT 24 ). To the DNA-immobilized surface, both the complementary (dA 20 ) and noncomplementary sequences (dT 20 ) were attached, with concentrations ranging from 100 fM to 1 μM, in 10-fold serial dilutions. The injection volumes of all the samples were <2 μl. The fluorescent intensity shown in Fig. 3b was obtained in the above-mentioned manner. Detection of influenza strain on carboxylic acid–SAM Cultured A/Udorn/307/1972 (H3N2) supplied from Nihon University was tested. Sensing surfaces coated with Au overlays using the evaporation method were incubated with 0.1 mM carboxylic acid–SAM formation reagent (Dojindo Laboratories, Japan) in absolute ethanolic solution for 3 h at room temperature with shaking. The SAM formed over the entire surfaces of the 35-mm-long channels. Then, the COOH-coated surface was washed thoroughly with copious volumes of absolute ethanol and dried under N 2 gas. This surface was treated with an equal volume of 100 mM N -hydroxysuccinimide (NHS) and 1-ethyl-3-(3-dimethylaminopropyl)carbodiimide hydrochloride (EDC; Biacore, Sweden) for 30 min at room temperature. Then, a plate seal was attached to the chip. Different numbers of haemagglutination units (HA units) of A/Udorn/307/1972 were immobilized onto these surfaces. The HA units for each experiment were determined as described previously [32] , where one HA unit is defined as the quantity of virus contained in 1 ml of a virus suspension of HA titre 1. The remaining free sites were blocked with 1 M ethanolamine (Biacore, Sweden). After blocking and washing, the rabbit IgG anti-influenza antibody (anti-A/Udorn/307/1972 antibody, 100 nM) was immobilized. The washing steps were performed with PBS, and detection was carried out by using 10 nM Alexa-Fluor-700-conjugated anti-rabbit antibody. Similarly, another influenza viral sample of H3N2 (A/Brisbane/10/2007; Prospec-Tany TechnoGene Ltd., Israel) and recombinant haemagglutinin from influenza H5N1 (A/chicken/India/NIV33487/2006; Sino Biological Inc., China) and H1N1 (A/California/07/2009; Sino Biological Inc., China) with 2,000 HA units ml −1 were tested against the anti-A/Udorn/307/1972 antibody. The injection volumes of all the influenza samples were <2 μl. Each fluorescent intensity shown in Fig. 4b,c was obtained in the manner described in the section above. How to cite this article: Nomura, K-i. et al. An angular fluidic channel for prism-free surface-plasmon-assisted fluorescence capturing. Nat. Commun. 4:2855 doi: 10.1038/ncomms3855 (2013).